Split-ball resonator as a three-dimensional analogue of planar split-rings Split-ring resonators are basic elements of metamaterials, which can induce a magnetic response in metallic nanosctructures. Tunability of such response up to the visible frequency range is still a challenge. Here we introduce the concept of the split-ball resonator and demonstrate the strong magnetic response in the visible for both gold and silver spherical plasmonic nanoparticles with nanometre scale cuts. We realize this concept experimentally by employing the laser-induced transfer method to produce near-perfect metallic spheres and helium ion beam milling to make cuts with the clean straight sidewalls and nanometre resolution. The magnetic resonance is observed at 600 nm in gold and at 565 nm in silver nanoparticles. This method can be applied to the structuring of arbitrary three-dimensional features on the surface of nanoscale resonators. It provides new ways for engineering hybrid resonant modes and ultra-high near-field enhancement. One of the main challenges in the field of plasmonics and metamaterials during the last decade is to engineer nanostructures with strong magnetic and electric dipole resonances at optical frequencies [1] , [2] , [3] , [4] , [5] . Getting these two resonances together in the same frequency range can lead to unique material properties associated with near-zero or even negative effective refractive index. The concept of the split-ring resonator (SRR), which provides a strong magnetic dipole response of metallic structures, was theoretically introduced by Pendry et al. [6] in 1999. Since then, many efforts to experimentally demonstrate a magnetic resonance of metallic structures have been reported, first in the gigahertz range [7] , then in the terahertz range [8] , and finally at optical frequencies [9] , [10] . It has been shown that scaling down the size of the SRR linearly increases the magnetic resonance frequency. However, this linear dependence saturates close to the visible spectral range mainly due to non-ideality of plasmonic metals at these frequencies [10] , [11] . Further control of the resonance position is possible using optimization of the design of SRRs [12] , [13] . More advanced designs, such as cut-wire pairs [14] , [15] , fish-net structures [16] , [17] , and nanoparticle clusters [18] , [19] , have also been implemented to facilitate metamaterial fabrication and further increase their magnetic resonance frequency. However, until now there have been few experimental demonstrations of resonant magnetic response of metallic nanostructures in the visible spectrum [18] , [19] , [20] , [21] , [22] , [23] , [24] , [25] , [26] . Strong dissipative losses of plasmonic nanostructures in the visible spectral range significantly limit the possibilities of shifting the magnetic resonance to higher frequencies. These losses arise due to imperfections of the nanostructures at the sub-100 nm scale and intrinsic losses inherent to plasmonic metals in this frequency range. One of the peculiarities of the magnetic response of metallic nanostructures is its possible overlap with a strong electric resonance provided by the same metallic elements. For example, it can be analytically demonstrated in the quasi-static limit that the magnetic dipole resonance of SRRs is always accompanied by the electric dipole resonance generated inside the gap of SRRs, being of the same or even higher order of magnitude [27] , [28] . Such combined electric and magnetic response of SRRs is appropriate to call an LC resonance to account for different multipolar modes contributing to the resonance peak. The use of low-loss resonant high-refractive index dielectric nanoparticles having strong Mie resonances of both electric and magnetic origins [29] , [30] , [31] , [32] , [33] , [34] , [35] can partially solve this problem and shift the magnetic resonance frequency to the blue spectral range [29] , [31] , [34] . In this case, a pure magnetic dipole resonance with very minor influence of other multipolar modes can be generated. In this Article, we introduce and experimentally demonstrate a new concept of a strong magnetic dipole resonance tuneable almost throughout the whole visible spectral range using standard plasmonic metals such as gold and silver. The key aspect is a nanometre-size cut fabricated inside an almost perfectly spherical plasmonic nanoparticle. Such a three-dimensional (3D) spherical design allows for shifting of the LC-type magnetic resonance down to the main electric dipole resonance wavelength in the visible spectral range. Partial contribution of different multipolar modes into the resonant scattering is analysed and strong magnetic dipole contribution is demonstrated. Experimentally, this novel design is realized by combining the almost perfect spherical nanoparticles achievable with the laser-induced transfer method (LIT) with the unprecedented patterning fidelity at nanometre scale dimensions characteristic of milling with a focused helium ion beam. Towards the understanding of the physics of such nanostructures, near-field enhancement and Poynting vector flow around them are also discussed. Numerical simulations A schematic representation of a metallic sphere with a cut, split-ball resonator (SBR), is shown in Fig. 1 . The nanocut is introduced on top of the sphere making it similar to 3D upright SRRs [36] , [37] . In this case, the coupling of light to the magnetic resonance mode should be more efficient due to both electric and magnetic field contributions. 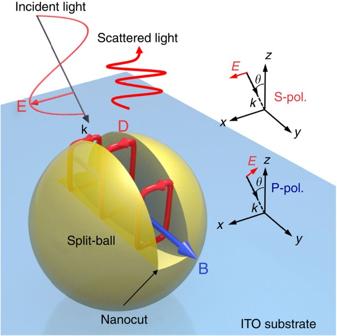Figure 1: Schematic representation of the SBR and geometry of spectral measurements. The nanocut is introduced on top of the metallic sphere. The incident light is directed onto the SBR from one side facing the nanocut at an angle of 58.5° to the surface normal. Two incident light polarizations are studied: s (perpendicular) and p (parallel) to the nanocut plane. The scattered light is collected from top by a microscope objective lens with 0.55 NA. Figure 1: Schematic representation of the SBR and geometry of spectral measurements. The nanocut is introduced on top of the metallic sphere. The incident light is directed onto the SBR from one side facing the nanocut at an angle of 58.5° to the surface normal. Two incident light polarizations are studied: s (perpendicular) and p (parallel) to the nanocut plane. The scattered light is collected from top by a microscope objective lens with 0.55 NA. Full size image To analyse the ability of the SBR to support the magnetic dipole resonance, we performed numerical simulations of its optical spectral properties using commercial CST Microwave Studio software. Results are shown in Fig. 2 for a gold sphere with diameter of 200 nm having a 50 nm wide cut going down to the centre of the sphere. The nanostructure is located in free space and excited by a plane wave directed from the top (antiparallel to z axis) with two different polarizations, parallel (along y axis) and perpendicular (along x axis) to the nanocut direction. Total scattering and absorption efficiencies by the nanostructure are shown in Fig. 2a (see Methods for details). 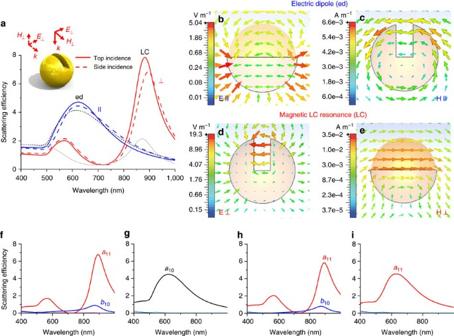Figure 2: Numerical simulations of optical properties of SBRs. (a) Total scattering efficiencies of an SBR formed by a 200 nm gold sphere with a 50 nm wide by 100 nm deep cut. The SBR is excited by a plane wave directed from top antiparallel tozaxis (solid curves) or from the side facing the cut alongyaxis (dashed curves). Polarization of the incident light is perpendicular or parallel to the cut. The black dotted curve represents scattering efficiency of the same particle without a cut. The grey curve is the absorption efficiency of the SBR for top excitation with polarization perpendicular to the cut. Inset is the schematic illustration of the SBR and directions of the incident plane waves. (b–e) Distributions of electric (b,d) and magnetic (c,e) field around the SBR at electric (b,c) (622 nm, polarization is parallel to the cut) and LC (d,e) (882 nm, polarization is perpendicular to the cut) resonance wavelengths. (f–i) Decomposition of the scattered field of SBR into multipole moments based on the vector spherical harmonics. SBR is excited from the top (f,g) or from the side facing the nanocut (h,i). Incident light polarization is perpendicular (f,h) or parallel (g,i) to the cut. All the electric and magnetic spherical multipole harmonics of the first and the second order are calculated and plotted in the figure. Only harmonics that have a noticable contribution are marked by corresponding coefficients (b10-magnetic dipole,a10anda11-electric dipoles).a11in all plots stays for a sum ofa11anda1-1mode contributions. Figure 2: Numerical simulations of optical properties of SBRs. ( a ) Total scattering efficiencies of an SBR formed by a 200 nm gold sphere with a 50 nm wide by 100 nm deep cut. The SBR is excited by a plane wave directed from top antiparallel to z axis (solid curves) or from the side facing the cut along y axis (dashed curves). Polarization of the incident light is perpendicular or parallel to the cut. The black dotted curve represents scattering efficiency of the same particle without a cut. The grey curve is the absorption efficiency of the SBR for top excitation with polarization perpendicular to the cut. Inset is the schematic illustration of the SBR and directions of the incident plane waves. ( b – e ) Distributions of electric ( b , d ) and magnetic ( c , e ) field around the SBR at electric ( b , c ) (622 nm, polarization is parallel to the cut) and LC ( d , e ) (882 nm, polarization is perpendicular to the cut) resonance wavelengths. ( f – i ) Decomposition of the scattered field of SBR into multipole moments based on the vector spherical harmonics. SBR is excited from the top ( f , g ) or from the side facing the nanocut ( h , i ). Incident light polarization is perpendicular ( f , h ) or parallel ( g , i ) to the cut. All the electric and magnetic spherical multipole harmonics of the first and the second order are calculated and plotted in the figure. Only harmonics that have a noticable contribution are marked by corresponding coefficients ( b 10 -magnetic dipole, a 10 and a 11 -electric dipoles). a 11 in all plots stays for a sum of a 11 and a 1-1 mode contributions. Full size image When the incident light polarization is parallel to the cut, only a single electric dipole resonance is excited inside the SBR, similar to a spherical nanoparticle without a cut ( Fig. 2a ). The electric dipole nature of this resonant peak is confirmed by electric and magnetic field distribution at the resonance wavelength ( Fig. 2b,c ) and decomposition of the near-field into spherical multipoles ( Fig. 2g , see detailed discussions below). When incident light polarization is perpendicular to the cut, two resonant peaks appear in the scattering spectrum: the first weaker peak is close to the position of the electric resonance, and the second, much stronger peak is at the longer wavelengths (see Fig. 2a ). This second resonant peak corresponds to the so-called LC resonance excited in the SBR similar to the case of SRRs [6] , [7] , [8] , [9] , [10] , [11] , [12] , [13] , [28] . The scattering intensity at this resonance is defined by a combination of strong electric and magnetic dipole contributions ( Fig. 2f , see detailed discussions below). The electric field at this resonant wavelength is strongly enhanced inside the cut generating circulating electric currents flowing around the nanocut inside the nanoparticle ( Fig. 2d ). On the other hand, the magnetic field is strongly enhanced and oscillates inside the nanocut parallel to its axis ( Fig. 2e ). Similar spectral behaviour can also be observed in the SBR excited from the side facing the nanocut (along y axis) with light polarization parallel (along z axis) and perpendicular (along x axis) to the cut ( Fig. 2a , dashed lines). Intensities and spectral positions of both electric and magnetic LC resonances in this case are almost unchanged compared with the case of excitation from the top. This shows that the magnetic response of SBRs is almost independent of the direction of incidence when it is varied in the nanocut plane ( yz ) and the incident light polarization is perpendicular to the gap. This property is similar to conventional SRRs, and it can be advantageous compared with multi-layer fishnets and stripes for a design of isotropic metamaterials. To understand better the nature of resonances excited inside the SBR for both polarizations, we perform a decomposition of the scattered field of the nanostructure into multipole moments based on the vector spherical harmonics [28] , [38] , [39] (see Methods for details). Results of this analysis for different incident angles and light polarizations are presented in Fig. 2f–i . Notation b 10 corresponds to the magnetic dipole mode, while a 10 and a 11 correspond to the electric dipole modes of two different types. For the incident light polarization parallel to the nanocut, only a single electric dipole resonant mode is excited while the excitation of other modes is negligibly small ( Fig. 2g,i ). This conclusion fully supports our previous discussion based on the electric and magnetic field distributions inside the SBR ( Fig. 2b,c ). We note here that the type of the electric mode changes for different polarizations from a 10 for incidence from the top ( Fig. 2g ) to a 11 , for incidence from the side ( Fig. 2i ) of the SBR. For polarization perpendicular to the nanocut, the resonance around 900 nm exhibits an enhancement of the magnetic dipole response b 10 for both incident angles (see Fig. 2f,h ). However, the electric dipole mode a 11 is also resonantly excited at this wavelength that is caused by a strong electric field enhancement inside the nanocut (see Fig. 2d ). This situation differs strongly from resonant dielectric nanoparticles where a pure magnetic dipole mode can be excited [29] , [30] , [31] , [32] , [33] , [34] , [35] . However, it is similar to conventional SRRs, where electric field enhancement inside the gap contributes to the scattering [27] , [28] . The relative contribution from the magnetic dipole mode to the scattering efficiency at LC resonance with respect to the electric dipole mode in SBR is comparable with and even stronger than that for conventional SRRs [28] (see Fig. 3 ). 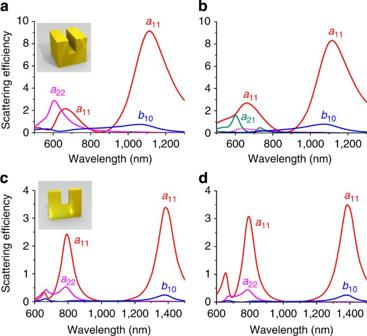Figure 3: Partial light scattering efficiencies by different spherical multipole modes excited inside different SRRs. (a,b) Scattering by a 3D gold cube with the gap on top. The cube dimentions are 200 × 200 × 200 nm3, the gap has the width of 50 nm and depth of 100 nm. The incoming plane wave is directed from top (a) and from the side facing the cut (b). (c,d) Scattering by a flat gold SRR standing upright. The SRR has dimensions of 200 × 200 × 20 nm3, the gap has the width of 50 nm and depth of 100 nm. The incoming plane wave is directed from top (c) and from the side facing the cut (d). All the electric and magnetic spherical multipole harmonics of the first and the second order are calculated and plotted in the figures. Only harmonics that have a noticable contribution are marked (a11-electric dipole,b10-magnetic dipole,a22anda21-electric quadrupoles). In casemis not zero,almin the plots stays for a sum ofalmandal-mmode contributions. Figure 3: Partial light scattering efficiencies by different spherical multipole modes excited inside different SRRs. ( a , b ) Scattering by a 3D gold cube with the gap on top. The cube dimentions are 200 × 200 × 200 nm 3 , the gap has the width of 50 nm and depth of 100 nm. The incoming plane wave is directed from top ( a ) and from the side facing the cut ( b ). ( c , d ) Scattering by a flat gold SRR standing upright. The SRR has dimensions of 200 × 200 × 20 nm 3 , the gap has the width of 50 nm and depth of 100 nm. The incoming plane wave is directed from top ( c ) and from the side facing the cut ( d ). All the electric and magnetic spherical multipole harmonics of the first and the second order are calculated and plotted in the figures. Only harmonics that have a noticable contribution are marked ( a 11 -electric dipole, b 10 -magnetic dipole, a 22 and a 21 -electric quadrupoles). In case m is not zero, a lm in the plots stays for a sum of a lm and a l-m mode contributions. Full size image In Fig. 3 , we also present the analysis of similar modes for light scattering by two SRR structures with the same size of the nanogap. One of the structures is a nanocube with the side length of 200 nm, gap width of 50 nm and depth of 100 nm, which is a 3D cubic analogue of the SBR ( Fig. 3a,b ). The second is a flat SRR obtained from the nanocube by reducing its width down to 20 nm ( Fig. 3c,d ). Both of the nanostructures exhibit an LC-type resonance at longer wavelengths, but with a smaller magnetic mode contribution compared with the SBR. The ratio of the maximum scattering efficiency by the magnetic dipole mode b 10 to the maximum scattering efficiency by the electric dipole mode a 11 is: 0.081 in Fig. 3a ; 0.095 in Fig. 3b ; 0.066 in Fig. 3c ; and 0.068 in Fig. 3d . These numbers are lower than the corresponding values for the SBR with a similar gap size: 0.13 in Fig. 2f and 0.14 in Fig. 2h . This means that the SBR supports a stronger magnetic dipole mode at LC-type resonance. It is also important to note that the relative contribution from the magnetic dipole to the LC resonance is somewhat higher in the 3D cube-like split-ring structure than in the flat SRR. This shows the advantage of 3D designs over flat nanostructures for generation of a strong magnetic dipole response. To show how both electric and magnetic resonances behave with respect to the cut parameters of the SBR, different cut depths have been simulated at a fixed cut width of 20 nm ( Fig. 4a ). The cut width has also been gradually changed at a fixed cut depth of 100 nm ( Fig. 4b ). As it is seen from the figures, both parameters strongly affects the LC resonance spectral position, while the position of the short-wavelength electric resonance is almost unchanged although its intensity is affected. When the cut depth is decreased, the LC resonance is blue-shifted, reaching the electric resonance position in the visible spectral range ( Fig. 4a ). This can be explained by a decrease of the capacitance of the gap ( C ) leading to an increase of the resonance frequency ( ω 2 =1/ LC ) that is in line with the SRRs theory [9] , [10] , [11] . On the other hand, decreasing of the width of the gap increases the gap capacitance, which leads to a decrease of the resonance frequency and a corresponding red-shift of the LC resonance peak ( Fig. 4b ). In both these cases, the inductance ( L ) changes slowly due to the large size of the sphere compared with the gap size. One should also note that the above LC circuit model initially developed for large SRRs is not fully applicable to our case of very small nanoparticles with nanocuts and is only used here as a simple illustration of the observed effects. Similar behaviour with respect to the depth of the gap has been observed earlier in flat split-ring resonators fabricated by focused ion beam milling of thin gold films [12] . It was shown that by controlling the depth of the gap, it is possible to shift the LC resonance down to the electric resonance wavelength. However, as the structures were flat, the position of both resonances was in the near-IR spectral range. In our case, the electric resonance position of the spherical particles is located in the visible spectrum that gives a possibility to shift the magnetic LC resonance down to visible wavelengths. 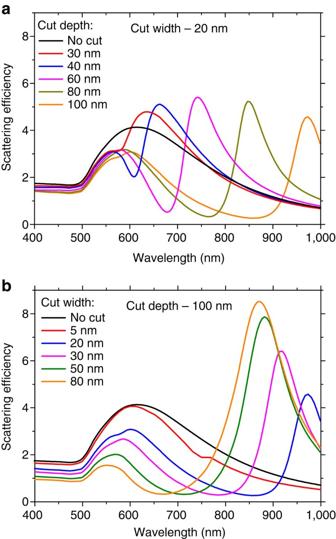Figure 4: Scattering properties of the SBR with varied cut parameters. The dependence of the scattering efficiency of the SBR on (a) the cut depth for a fixed cut width of 20 nm and (b) on the cut width at a fixed cut depth of 100 nm. The incident plane wave is directed from top of the SBR with light polarization perpendicular to the cut. The gold sphere diameter is 200 nm. Figure 4: Scattering properties of the SBR with varied cut parameters. The dependence of the scattering efficiency of the SBR on ( a ) the cut depth for a fixed cut width of 20 nm and ( b ) on the cut width at a fixed cut depth of 100 nm. The incident plane wave is directed from top of the SBR with light polarization perpendicular to the cut. The gold sphere diameter is 200 nm. Full size image Experiment To verify this concept experimentally, we first fabricated gold and silver nanoparticles using the LIT in combination with e-beam lithography [40] (see Methods for more details). This method allows producing nanoparticles with almost perfect spherical shape and high surface quality. The size of the nanoparticles is controlled using an initial lithography step while their spherical shape and low surface roughness is assured by strong surface tension forces of molten metal during the laser processing. Then nanocuts with straight sidewalls have been produced on top of the nanoparticles using focused helium (He) ion beam milling. In comparison with standard FIB systems [41] , [42] that use gallium (Ga) ions, helium ion microscope (HIM) can provide significantly higher structuring resolution [43] , [44] , [45] . Also, in contrast to standard gallium-ion based FIB systems, HIM does not significantly dope the sidewalls of the materials during milling and thus may retain good plasmonic properties of the nanoparticles [41] , [46] . HIM images of two gold nanoparticles with cuts fabricated by this combined method are shown in Fig. 5a,b . These nanoparticles have a similar diameter of around 170 nm and cut width of around 15 nm. The structured cut can be controlled in depth and width (down to <5 nm) but in this case was varied to match the modelling predictions. Variable depth was achieved by varying the dwell time at a fixed beam current. The dwell time was 25% longer for the particle shown in Fig. 5a compared with that shown in Fig. 5b , which resulted in a deeper cut (see Methods for details). Optical properties of these nanoparticles have been studied using a single-nanoparticle spectroscopy setup [31] . Measurements were performed in dark field geometry with illumination from one side facing the nanocut ( k vector is in the yz plane). Two different polarizations of excitation source have been studied: parallel and perpendicular to the nanocut (see Fig. 1 and Methods for details). In this excitation geometry, p-polarization (lying in the yz plane) should only couple to the electric dipole resonance of the sphere while s-polarization (along x axis) should excite both electric and magnetic dipoles. Results of these measurements for the two gold particles are shown in Fig. 5c,d . For p-polarization, which is parallel to the cut, only a single scattering peak corresponding to the electric dipole resonance of the sphere is observed. For s-polarization, two resonances are detected, LC resonance on the long wavelength side and a leftover of the electric dipole on the short-wavelength side. For the particle with a deeper cut ( Fig. 5a,c ), the LC resonance position is red-shifted compared with the particle with a shallower cut ( Fig. 5b,d ). These results are in a very good agreement with theoretical predictions discussed in the previous section ( Fig. 4a ). To the best of our knowledge, the wavelength of magnetic resonance of 600 nm obtained for the gold SBR in Fig. 5b,d is the shortest compared with all gold-based nanostructures reported so far. 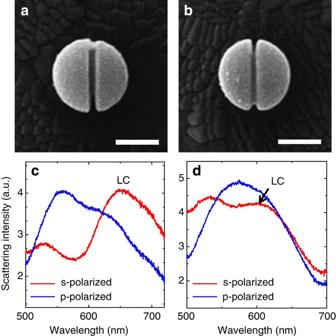Figure 5: Experimental realization of gold SBRs. (a,b) HIM images of two gold nanoparticles with similar diameters of 170 nm and cuts width of 15 nm. Cut depth in (a) is larger than in (b), which is obtained by 25% longer helium ion beam milling time. Scale bars correspond to 100 nm. (c,d) Scattering spectra of the particles shown in (a,b) for incident light with s (perpendicular to the cut) and p (parallel to the cut) polarizations. LC labels show spectral position of the LC resonance. It is observed at 650 nm in (c) and 600 nm in (d). Figure 5: Experimental realization of gold SBRs. ( a , b ) HIM images of two gold nanoparticles with similar diameters of 170 nm and cuts width of 15 nm. Cut depth in ( a ) is larger than in ( b ), which is obtained by 25% longer helium ion beam milling time. Scale bars correspond to 100 nm. ( c , d ) Scattering spectra of the particles shown in ( a , b ) for incident light with s (perpendicular to the cut) and p (parallel to the cut) polarizations. LC labels show spectral position of the LC resonance. It is observed at 650 nm in ( c ) and 600 nm in ( d ). Full size image To show that this concept may also work at even shorter wavelengths, the same approach has been applied to fabricate SBRs made of silver. Plasmonic resonance of silver nanoparticles is blue-shifted compared with gold. Thus one may expect further blue-shift of the magnetic resonance position in silver SBRs. Results for silver are shown in Fig. 6 . First, a silver SBR has been fabricated with a particle diameter of around 170 nm and a cut width of around 15 nm that is similar to the gold SBRs discussed earlier ( Fig. 6a ). The LC resonance position in this case is around 640 nm ( Fig. 6d ) that is similar to the above results for gold nanoparticles. However, this resonance is more pronounced and well separated from the electric dipole resonance located around 500 nm. To further shift both resonances to shorter wavelengths, a smaller silver nanoparticle with a diameter of around 80 nm and a 12 nm wide cut has been fabricated ( Fig. 6b ). In this case, the LC resonance position is further blue-shifted reaching the wavelength of 570 nm, which is significantly smaller than earlier reported results obtained with SRRs [10] , [11] , [12] , [13] and coupled nanoparticles [18] , [19] and is comparable with the best results obtained with multi-layer stripes and fishnets [21] , [22] . However, in contrast to the stripes, fishnets and other multi-layer structures whose magnetic response can only be obtained under a single excitation direction, SBRs (similar to SRRs) possess a strong magnetic response for all incident directions lying in the plane parallel to the nanocut that may hold a bigger promise for metamaterial design and fabrication. 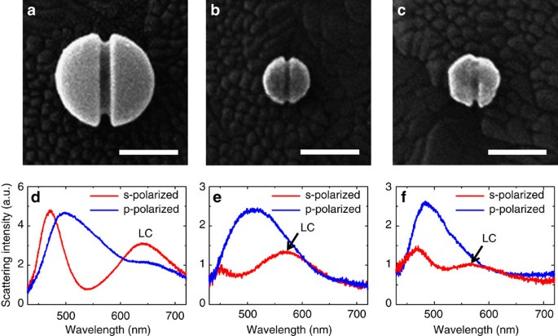Figure 6: Experimental realization of silver SBRs. (a–c) HIM images of three silver nanoparticles with diameters of 170 nm (a) and 80 nm (b,c) and a cut width of 15 nm (a) and 12 nm (b,c). The nanoparticles in (a,b) are produced by the LIT method whereas the nanoparticle in (c) is chemically synthesized. Scale bars correspond to 100 nm. (d–f) Scattering spectra of the nanoparticles shown in (a–c) for incident light with s (perpendicular to the cut) and p (parallel to the cut) polarizations. LC labels show spectral position of the LC resonance. It is observed at 640 nm in (d), 570 nm in (e) and 565 nm in (f). Figure 6: Experimental realization of silver SBRs. ( a – c ) HIM images of three silver nanoparticles with diameters of 170 nm ( a ) and 80 nm ( b , c ) and a cut width of 15 nm ( a ) and 12 nm ( b , c ). The nanoparticles in ( a , b ) are produced by the LIT method whereas the nanoparticle in ( c ) is chemically synthesized. Scale bars correspond to 100 nm. ( d – f ) Scattering spectra of the nanoparticles shown in ( a – c ) for incident light with s (perpendicular to the cut) and p (parallel to the cut) polarizations. LC labels show spectral position of the LC resonance. It is observed at 640 nm in ( d ), 570 nm in ( e ) and 565 nm in ( f ). Full size image To show how the surface quality of the nanoparticles influences their resonant properties, HIM cut have also been introduced into a commercial chemically synthesized silver nanoparticle (NanoComposix) of 80 nm size ( Fig. 6c,f ). In this case, the electric resonance position is further blue-shifted, which may probably be explained by a higher crystallinity of the chemically synthesized silver nanoparticles. However, the LC resonance is less pronounced due to the inferior surface quality of these nanoparticles compared with the nanoparticles obtained by LIT method. Finally, light energy flow inside and outside the SBR at the magnetic resonance wavelength has been simulated by CST Microwave Studio software. This study is useful to understand the high scattering and absorption efficiencies of the nanostructures. Similar SBR parameters as in Fig. 2 have been used in these simulations. The Poynting vector lines at the LC resonance wavelength of 882 nm are shown in Fig. 7a,b in two different cross-section planes. The colour map corresponds to the distribution of the modulus of the Pointing vector. It is seen in Fig. 7a that in the xz plane, the Poynting vector lines spanning an area exceeding the nanoparticle cross-section by several times are collected and concentrated inside the nanocut. This generates significant field enhancement of the order of 20 inside the cut. Similar simulations performed for a silver SBR with diameter of 170 nm and a cut width of 15 nm (similar to the one shown in Fig. 6a ) demonstrate even larger field enhancement inside the cut around 45 (not shown here). This energy flow passing the cut does not come out of the SBR forming optical vortices from both sides of the nanostructure. This explains the strong absorption resonance at this wavelength. On the other hand, in the yz plane, most of the Poynting vector lines are strongly deviated and pass around the SBR without penetrating into it, resulting in a strong scattering efficiency at the LC resonance. Figure 2c shows the separatrix absorption surface of the SBR in the xy plane. All Poynting vector lines inside the separatrix surface go into the SBR and are absorbed [47] , [48] . Strong asymmetry of the separatrix surface in x and y directions support our discussion above. 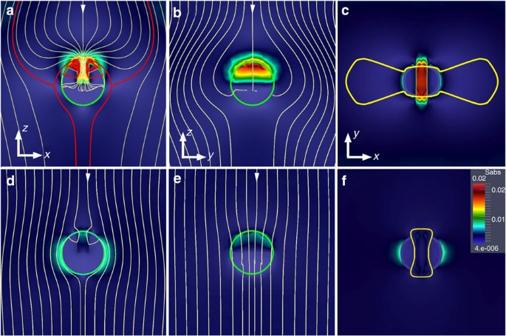Figure 7: Poynting vector distribution around gold SBR. (a–c) at LC resonance wavelength of 882 nm, (d–f) at minimum scattering wavelength of 710 nm. (a,d) showxzcross-section plane in the middle of the sphere. (b,e) showyzcross-section plane in the middle of the sphere. (c,f) show separatrix absorption surfaces (limited by yellow separatrix lines) of the SBR inxycross-section plane. The SBR has 200 nm diameter and a cut with 50 nm width and 100 nm depth (similar toFig. 2). Colour map represents distribution of the modulus of the Poynting vector around the nanoparticle. Red lines show separatrices of the energy flow47,48. Green circles highlight the nanoparticle location. Figure 7: Poynting vector distribution around gold SBR. ( a – c ) at LC resonance wavelength of 882 nm, ( d – f ) at minimum scattering wavelength of 710 nm. ( a , d ) show xz cross-section plane in the middle of the sphere. ( b , e ) show yz cross-section plane in the middle of the sphere. ( c , f ) show separatrix absorption surfaces (limited by yellow separatrix lines) of the SBR in xy cross-section plane. The SBR has 200 nm diameter and a cut with 50 nm width and 100 nm depth (similar to Fig. 2 ). Colour map represents distribution of the modulus of the Poynting vector around the nanoparticle. Red lines show separatrices of the energy flow [47] , [48] . Green circles highlight the nanoparticle location. Full size image As a comparison, energy flow at the wavelength of the minimum scattering of 710 nm is also shown in the xz and yz planes in Fig. 7d,e , respectively. In this case, the Poynting vector lines pass through the SBR with only a very small absorption and scattering making the nanostructure almost invisible. The separatrix surface in this case ( Fig. 7f ) has a different geometry compared with the resonance ( Fig. 7c ) and is smaller than the geometrical cross-section of the particle. This behaviour is associated with destructive Fano-type interference between the electric dipole and LC resonance inside the SBR [18] , [49] , [50] , [51] . In conclusion, a novel concept to realize optical magnetism at visible frequencies with standard plasmonic materials such as gold and silver is proposed. This concept is based on a spherical nanoparticle with a precision patterned nanocut. Due to a volumetric 3D shape of the proposed design a strong magnetic response tunable through the visible spectral range can be obtained. Experimentally, this unique design has been realized using laser-induced melting of nanostructures to obtain near-perfect spherical nanoparticles and helium ion beam milling to make cuts with nanometre resolution and straight sidewalls. Magnetic resonance wavelength down to 600 nm for gold and 565 nm for silver has been experimentally demonstrated here, which corresponds and exceeds previous experimental results. This novel approach to engineer resonant modes of perfect spherical nanoparticles opens new possibilities to design novel nanostructures with unique modes and high field enhancement regions that may be promising for applications to metamaterials, surface-enhanced Raman scattering, heat-assisted magnetic recording, and nanoantennas. E-beam nanofabrication Gold and silver nanodisks with various diameters were fabricated on quartz substrates by electron beam lithography (Elonix 100KV EBL system). First, 120 nm positive resist (ZEP) was coated on the sample. After baking it at 180 °C for 2 min, a 20 nm Espacer was coated on the top of the resist to avoid a charging effect. The structural geometries were defined by electron beam in the resist followed by a standard development. Then a thin Ti film (2 nm thick) and a 50 nm thick Au or Ag layer were deposited on the substrate by e-beam evaporation. Ti film was evaporated to ensure good adhesion between the Au/Ag layers and the substrate. A lift-off procedure was the last step to generate the nanodisks. Laser processing Following the first nanofabrication steps, femtosecond laser irradiation has been applied to the nanostructures. In these experiments, commercial 1 kHz femtosecond laser system (Tsunami+Spitfire, Spectra Physics) delivering 1 mJ, 100 fs laser pulses at a central wavelength of 800 nm has been used. The laser beam with a diameter of 4 mm was directed onto a square-shaped pinhole with 300 μm size. The beam just after passing through the pinhole was imaged onto the sample surface using a × 20 long distance microscope objective (Mitutoyo, MPlan NIR 20) and a 200 mm focus tube lens. This image transfer results in a square shape 15 μm size flattop laser beam profile on the sample surface. The laser beam power was attenuated by a neutral glass filter (15%) and a half-wave plate+polarizer to get the fluence of around 0.5 J per cm 2 on the sample surface. The nanostructures have been melted by the laser irradiation, transformed into spherical nanodroplets by surface tension forces and transferred onto an ITO-coated glass substrate. After solidification, the molten droplets form almost perfect spherical nanoparticles. More details about the LIT and its application to nanostructures and continuous metal films for nanoparticle generation can be found in refs 40 , 52 , 53 , 54 . Helium ion beam milling The HIM (Zeiss Orion Plus) is capable of milling extremely high-resolution structures with lateral dimensions of less than 5 nm. When combined with a sophisticated pattern generator and custom writing strategies, near arbitrary control of the surface features is possible. In this work, the helium ion beam at a current of 0.5 pA with a landing energy of 35 kV in conjunction with a Nabity pattern generator was employed to further structure the surfaces of the fabricated nanoparticles. The ion fluence across the cut was varied and optimized with a multi-pass writing strategy to prevent over-milling at the edges, and eliminate residual metal redeposition while maintaining the pattern fidelity. The beam dwell time was modulated throughout the length of the cut, with commensurately longer milling time at the centre of the cut compared with the edges to compensate for the centre's increased metal thickness, as well as mitigate secondary effects such as decreased redeposition at the edges. For the gold particle in Fig. 5a , the ion fluence was about 5 × 10 16 ions per cm 2 at the edges with intermediate sections having a varying fluence of 7.5 × 10 17 , 3.25 × 10 18 , 5.25 × 10 18 and 6.75 × 10 18 ions per cm 2 towards the centre. The ion fluence was decreased by 20% for the particle in Fig. 5b . For the silver particle in Fig. 6a , the fluence at the edges was about 8 × 10 17 ions per cm 2 with intermediate sections having a varying fluence of 2.5 × 10 18 , 3.75 × 10 18 , 5 × 10 18 ions per cm 2 and 8 × 10 18 ions per cm 2 towards the centre. Silver particles in Fig. 6b,c were patterned with a fluence of 5 × 10 17 ions per cm 2 at the edges, 2.5 × 10 18 ions per cm 2 at the centre and a gradually increasing fluence of 1 × 10 18 , 1.5 × 10 18 and 2 × 10 18 ions per cm 2 in between. Single-nanoparticle spectroscopy Spectral analysis of the fabricated SBRs was performed using a single-nanoparticle spectroscopy setup (see ref. 31 for details) in dark field geometry ( Fig. 1 ). The sample was irradiated by a halogen lamp source from one side facing the nanocut at an angle of 58.5° to the surface normal (see ref. 34 for details of dark field spectral measurements). The scattering by the nanostructure has been collected from the top into a solid angle corresponding to the microscope objective lens with 0.55 NA. Two different incident light polarizations have been studied: s-polarization—perpendicular to the nanocut and parallel to the substrate surface, and p-polarization—parallel to the nanocut and at an angle to the substrate surface ( Fig. 1 ). The collected scattering spectra for both polarizations are normalized to the halogen lamp spectrum measured in bright-field transmission geometry. This normalization method provides correct shapes of the scattering spectra without keeping information on total scattering amplitudes. Theoretical and numerical analysis Numerical simulations of the SBRs were performed using commercial CST Microwave Studio software. Scattering and absorption efficiencies by the nanostructures were obtained by dividing the corresponding cross-sections by the overall geometrical cross-section of the nanoparticle. To calculate relative contributions of different modes excited inside the SBR, we perform a decomposition of the scattered field of the nanostructure into multipole moments based on the vector spherical harmonics [28] , [38] , [39] . To do that, we calculated electric a l-m and magnetic b lm multipole coefficients via the electric scattered field E s on a spherical surface enclosing the split ball centred at the origin (centre of the split ball) as follows: where R is the radius of the enclosing sphere, k is the wavevector, h l (1) is the Hankel function with the asymptotics of the outgoing spherical wave, E 0 is the amplitude of the incident wave, Y lm and X lm are scalar and vector spherical harmonics [39] . Based on these multipole coefficients, we can also calculate partial scattering efficiencies associated with a particular spherical harmonic where d is the outer radius of the split ball. The total scattering efficiency can be obtained by taking the full sum of all partial contributions: Although our system does not exhibit pure azimuthal symmetry, the numerical results demonstrate that mulitpole coefficients still hold the following relations: and that can be explained due to a relatively narrow nanocut in the split ball. Based on these results we can introduce the effective scattering efficiencies which are the sum of two contribution for ( l , m ) and ( l ,− m ) harmonics for m ≠0. These efficiencies were plotted in Fig. 2f–i for all electric and magnetic modes of the first and the second order (dipoles and quadrupoles). Electric and magnetic dipole modes, which have the strongest contribution to the total scattering, are marked in Fig. 2 as: b 10 -magnetic dipole mode, and a 10 and a 11 -electric dipole modes. How to cite this article : Kuznetsov, A. I. et al. Split-ball resonator as a three-dimensional analogue of planar split-rings. Nat. Commun. 5:3104 doi: 10.1038/ncomms4104 (2014).